Coupled reversion and stream-hyporheic exchange processes increase environmental persistence of trenbolone metabolites Existing regulatory frameworks for aquatic pollutants in the United States are idealized, often lacking mechanisms to account for contaminants characterized by (1) bioactivity of both the parent and transformation products and (2) reversible transformations (that is, metastable products) driven by chemical or physical heterogeneities. Here, we modelled a newly discovered product-to-parent reversion pathway for trenbolone acetate (TBA) metabolites. We show increased exposure to the primary metabolite, 17α-trenbolone (17α-TBOH), and elevated concentrations of the still-bioactive primary photoproduct hydroxylated 17α-TBOH, produced via phototransformation and then converted back to 17α-trenbolone in perpetually dark hyporheic zones that exchange continuously with surface water photic zones. The increased persistence equates to a greater potential hazard from parent-product joint bioactivity at locations and times when reversion is a dominant trenbolone fate pathway. Our study highlights uncertainties and vulnerabilities with current paradigms in risk characterization. With tens of thousands of synthetic chemicals discharged to the environment, it is unrealistic to individually collect comprehensive environmental fate data to accurately define human and ecological health risks. Accordingly, human and ecological risk assessments currently use approaches built upon expectations from the relatively small subset of contaminants whose environmental fates and associated biological risks are well understood. However, the danger implicit in this strategy is that prediction of presumptive biological risks can fail catastrophically for chemical contaminants with reactivities that deviate from expectations. To address this shortfall, computational and numerical modelling efforts can project the environmental fate of chemicals based on a combination of chemical properties and environmental system conditions. Such modelling also can be used to initially screen ecological risks and guide future research efforts such as field sampling. Especially for chemicals of high production volume, widespread environmental occurrence, or unusually high potency and potential toxicity, such efforts are critical to improving assessment of biological risk. As an example, we point to our recent research efforts on the product-to-parent reversion of trenbolone acetate (TBA) metabolites, a previously unidentified chemical process with a poorly understood influence on the environmental fate of these widely used and potent growth promoters [1] . The use of growth promoting steroid hormones is ubiquitous in the US beef cattle industry, with these pharmaceuticals reducing production costs by up to 7% and representing ∼ $1 billion annually in incremental economic value [2] . Administered by ear implantation, TBA is converted to the androgen 17β-trenbolone, which is far more potent than testosterone and primarily responsible for anabolic effects such as increased weight gain. 17β-trenbolone is excreted along with other TBA metabolites including 17α-TBOH and trendione that are subsequently mobilized in runoff ( Fig. 1 ) [3] . 17α-TBOH represents about 95% of identifiable excreted metabolites by mass [4] , although a number of unidentified TBA metabolites likely exist. Given the typical application rates of TBA to cattle, mass balance calculations predict that thousands of ng l −1 are possible in agricultural runoff [5] , [6] , although concentrations observed in receiving waters are typically far lower when detected [7] , [8] . Field observations have documented 1,700 ng l −1 17α-TBOH in manure lagoons [9] , and 55±22 ng g −1 in solid manure and surface soils [10] . TBA metabolite exposure is problematic for ecosystem health because 17α-TBOH and 17β-TBOH are potent endocrine disruptors, with exposure to as little as 10–30 ng l −1 significantly reducing fecundity, resulting in phenotypic sex reversal in fish, or altering endocrine function [11] , [12] , [13] . 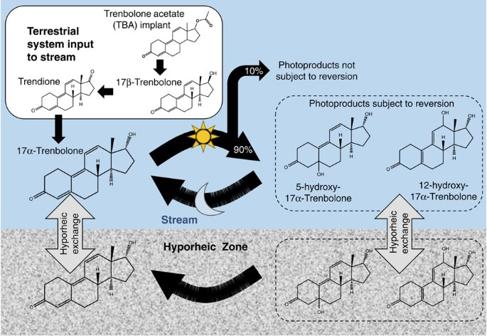Figure 1: Overview of interacting physical and chemical systems. Structures of TBA (primary component implanted into cattle), metabolites 17β-TBOH (pharmacologically active androgen), trendione, 17α-TBOH (primary product excreted to the environment) and 17α-TBOH photoproducts (5- and 12-hydroxy-17α-TBOH) that are subject to reversion under dark conditions. Figure 1: Overview of interacting physical and chemical systems. Structures of TBA (primary component implanted into cattle), metabolites 17β-TBOH (pharmacologically active androgen), trendione, 17α-TBOH (primary product excreted to the environment) and 17α-TBOH photoproducts (5- and 12-hydroxy-17α-TBOH) that are subject to reversion under dark conditions. Full size image Until recently, rapid photodegradation of TBA metabolites in sunlit surface waters was believed to effectively mitigate their environmental risk [14] . However, we recently reported that the major photoproducts of recognized TBA metabolites, hydroxylated trenbolone species (hereafter hydroxy-17α-TBOH), are metastable and able to regenerate their respective parent compounds [1] . These reversible transformations (that is, ‘product-to-parent reversion’) occur when the rapid forward reaction by direct photolysis (that is, photohydration) in sunlight is countered by slower dehydration reactions when dark (see overview of physical-chemical system in Fig. 1 ). The relative rates of the forward and reverse reactions ultimately control net photolysis or reversion as a function of both physical characteristics (for example, light exposure) and biogeochemical conditions (for example, pH, temperature). The first objective of this study is to quantify the impacts of these newly reported reversible reactions on TBA metabolite concentrations in fluvial systems. We designed a series of numerical experiments to highlight key differences between our former (without-reversion) and current (with-reversion) understanding of the environmental fate for TBA metabolites. We hypothesize that the net effect of these processes operating in stream-hyporheic systems is increased persistence of TBA metabolites in the stream system, resulting in enhanced hydraulic transport and higher concentrations. This increased persistence is particularly troublesome for compounds like TBA metabolites where both the parent species and transformation products retain bioactivity [15] . Our second objective is to characterize expected joint bioactivity (JBA) arising from the suite of TBA metabolites and their photoproducts, including their spatial and temporal occurrence, partitioning and interactions with hydrological dynamics in stream systems. Accordingly, we calculate JBA with- and without-reversion to estimate the risk represented by atypical characteristics like reversible transformation processes, and extend our findings to consider a broader range of risk, wherein JBA is a blend of product and parent concentrations with different relative potencies. This work extends the concept of ‘joint persistence’ originated by Fenner et al . [16] , [17] , [18] to account for the range of potencies (that is, bioactivity metrics) expected for parent compounds and related transformation products. We note that, although our simulations are based on TBA metabolites as the pollutant of interest, they are applicable to a range of compounds for which reversible transformations driven by interacting, heterogeneous physical and/or chemical processes occur in the environment. Our results demonstrate that interactions of primarily physical and chemical processes can yield unexpected transport and fate behaviours, ultimately retaining a substantial fraction of TBA-derived potency in the system over many days. Finally, we generalize model results for cases where differential reactivity controls parent-product partitioning and JBA in the system. Although this modelling effort focuses on an idealized case for the transport and fate of TBA metabolites to better understand the environmental implications of their reversion pathway, results are applicable more generally to any system where heterogeneity in the physical or chemical system affects parent-product fate dynamics. Ultimately, we demonstrate that current assessment approaches remain prone to unintended consequences because they are ill-equipped for pollutants with atypical transformation pathways and they cannot accurately predict how heterogeneous physical and chemical environments control JBA. Reversion increases 17α-TBOH persistence in stream networks The numerical simulations demonstrate that reversion cycling increases in-stream and hyporheic 17α-TBOH concentrations compared with the without-reversion case throughout the stream network ( Fig. 2 ). Spatial profiles for cases with- and without-reversion are shown for both 17α-TBOH and hydroxy-17α-TBOH throughout a 24-hr cycle in Fig. 2 (see also Supplementary Movie 1 , Supplementary Fig. 1 ). The spatial and temporal scales to achieve removal of peak concentrations during a 24-hour cycle as the management target of interest vary between cases (maximum of shaded 24-hour range for 17α-TBOH; Fig. 3 ). Advective travel times to achieve 50% removal of input concentrations are 14.4 and 13.8 h (38.0 and 36.2 km) for the cases with- and without-reversion, respectively. Times to 90% removal are 287.4 and 16.2 h (757.4 and 42.7 km) for with- and without-reversion cases, respectively, and the disparity grows to 406.9 and 25.9 h (1,072.4 and 68.2 km) to achieve 99% removal (linear extrapolation beyond the model domain for the with-reversion case). In contrast, timescales for the forward reaction in idealized laboratory studies were reported as 1.1 to 2.5 h. In our simulations, the complexity of the fluvial environment—particularly the perpetually-dark hyporheic zone where reversion processes would dominate even during periods of light—results in the increased persistence of 17α-TBOH in the stream. 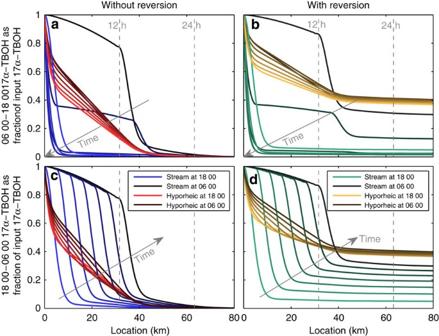Figure 2: Spatial profiles of 17α-TBOH through a 24-hour cycle. Spatial profiles for 17α-TBOH without (left column) and with (right column) product-to-parent reversion. Profiles are shown through a typical 24-hour cycle divided into periods of daylight (top row, 0600–1800 hours) and darkness (bottom row, 1,800–0,600 hours), with individual profiles at 2-hour intervals. Vertical dashed lines indicate distances for 12 and 24 h of downstream advection in the stream channel. Concentration profiles reflect the interaction of physical transport processes (primarily advection, hyporheic exchange) with chemical processes (time-variable photolysis, persistent reversion). The stream profile is dominated by advection of the input concetrations of 17α-TBOH during periods of darkness (bottom row) and by photolysis during periods of light (top row). Reversion of hydroxy-17α-TBOH to 17α-TBOH increases hyporheic concentrations throughout the domain, particularly at distances downstream of about 10 km. Figure 2: Spatial profiles of 17α-TBOH through a 24-hour cycle. Spatial profiles for 17α-TBOH without (left column) and with (right column) product-to-parent reversion. Profiles are shown through a typical 24-hour cycle divided into periods of daylight (top row, 0600–1800 hours) and darkness (bottom row, 1,800–0,600 hours), with individual profiles at 2-hour intervals. Vertical dashed lines indicate distances for 12 and 24 h of downstream advection in the stream channel. Concentration profiles reflect the interaction of physical transport processes (primarily advection, hyporheic exchange) with chemical processes (time-variable photolysis, persistent reversion). The stream profile is dominated by advection of the input concetrations of 17α-TBOH during periods of darkness (bottom row) and by photolysis during periods of light (top row). Reversion of hydroxy-17α-TBOH to 17α-TBOH increases hyporheic concentrations throughout the domain, particularly at distances downstream of about 10 km. 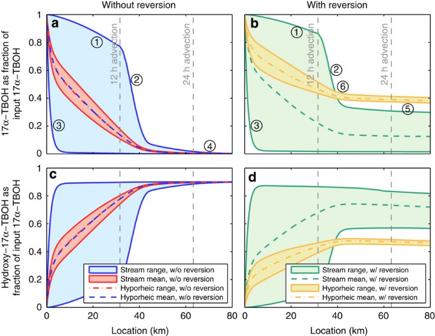Figure 3: Twenty-four-hour average, maximum and minimum 17α-TBOH and hydroxy-17α-TBOH concentrations. Twenty-four-hour average concentrations (dashed lines) and ranges (shaded regions) for 17α-TBOH and hydroxy-17α-TBOH in the stream-hyporheic system through a typical 24-hour cycle at dynamic steady state. Vertical dashed lines indicate distances for 12 and 24 h of downstream advection in the stream channel. Labels indicate (1) advection of input concentration in-stream during period of darkness; (2) rapid photolysis of 17α-TBOH advected during night time period, decay is not exponential because the forward reaction rate is time-variable with solar loading; (3) rapid photolysis of 17α-TBOH input during daylight period; (4) 99% removal of 17α-TBOH achieved after 25.9 h; (5) equilibrium of photolysis and reversion, linear decay due to partitioning of 10% of forward reaction of 17α-TBOH to non-revertible products; and (6) hyporheic zone has only a source function downstream of 38 km. Full size image Figure 3: Twenty-four-hour average, maximum and minimum 17α-TBOH and hydroxy-17α-TBOH concentrations. Twenty-four-hour average concentrations (dashed lines) and ranges (shaded regions) for 17α-TBOH and hydroxy-17α-TBOH in the stream-hyporheic system through a typical 24-hour cycle at dynamic steady state. Vertical dashed lines indicate distances for 12 and 24 h of downstream advection in the stream channel. Labels indicate (1) advection of input concentration in-stream during period of darkness; (2) rapid photolysis of 17α-TBOH advected during night time period, decay is not exponential because the forward reaction rate is time-variable with solar loading; (3) rapid photolysis of 17α-TBOH input during daylight period; (4) 99% removal of 17α-TBOH achieved after 25.9 h; (5) equilibrium of photolysis and reversion, linear decay due to partitioning of 10% of forward reaction of 17α-TBOH to non-revertible products; and (6) hyporheic zone has only a source function downstream of 38 km. Full size image Patterns of 17α-TBOH are spatially and temporally variable in the stream network. At night, the inflowing 17α-TBOH is primarily advected in the stream channel. Hyporheic exchange decreases maximum in-stream concentrations of 17α-TBOH due to exchange between the relatively high concentration stream water and the low concentration hyporheic water in both with- and without-reversion cases ( Fig. 3(1) ). The decrease is more pronounced in the without-reversion case, where concentration gradients between the stream and hyporheic zone are steeper (hyporheic reversion to 17α-TBOH decreases this gradient in the with-reversion case). The results in Fig. 3 provide data that could be used to estimate both acute and chronic exposure, best characterized by the maximum and mean concentrations, respectively. After 12 h of advection, maximum in-stream concentrations are 77.1 and 86.3% of the input concentration for the without-reversion and with-reversion cases, respectively. When forward photolysis rates exceed reversion rates (during periods of light), rapid decreases of in-stream 17α-TBOH concentrations occur in both cases ( Fig. 3(2) ). In-stream 24 h minimum values are dominated by the forward photolysis reaction ( Fig. 3(3) ), achieving initial removals of 50 and 90% at 0.34 and 1.20 h for the without-reversion case, and 0.35 and 1.24 h for the with-reversion case. Removal of 99% of the input 17α-TBOH is achieved for the without-reversion case after 25.9 h ( Fig. 3(4) ), while daily peak 17α-TBOH concentrations of 30.4 and 40.9% persist in the stream and hyporheic zone, respectively ( Fig. 3(5) ). Finally, beyond 38 km in the network, hyporheic zone concentrations of 17α-TBOH are higher than in-stream concentrations throughout a complete 24 h cycle ( Fig. 3(6) ). Upstream of this location, hyporheic concentrations oscillate between being higher and lower than in-stream concentrations. This location defines a transition point from an upstream source-dominated reach to a downstream reversion-dominated reach. The transition location is primarily set by in-stream advection and photoperiod, specifically the distance 17α-TBOH is transported during periods where the reversion rate exceeds the photolysis rate. Longer photoperiods or slower advective velocities move this location closer to the source. In these cases, the partitioning between the stream and hyporheic zone, responsible for the declining maximum concentrations in-stream ( Figs 2 , 3 , 4 ), decreases in importance. 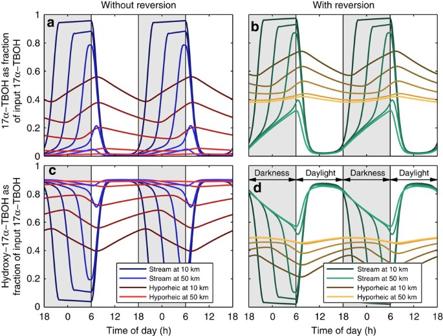Figure 4: Time series of in-stream and hyporheic 17α-TBOH and hydroxy-17α-TBOH concentration at selected spatial locations. Time series of stream and hyporheic concentrations for 17α-TBOH without (left column) and with (right-column) product-to-parent reversion at selected locations. Two typical 24 h cycles are presented for each spatial location. Grey and white shaded regions indicate periods of darkness (reversion dominance in the stream) and daylight (photolysis dominance in the stream), respectively. For cases without-reversion, hyporheic zones alternate between net sources of 17α-TBOH to the stream. The hyporheic zone is a net source of 17α-TBOH when stream concentration is less than hyporheic concentration (that is, during daylight periods when photolysis dominates in the stream). Hyporheic zones are a net sink for in-stream 17α-TBOH when the stream concentration is greater than the hyporheic concentration (typically during periods of darkness). Cases with and without-reversion have similar source-sink behaviour for the first 38 km of transport, but hyporheic zones become persistent sources of 17α-TBOH to the stream beyond this location. In these downstream locations, hyporheic reversion is able to increase in-stream concentrations to nearly 40% of their input concentration in some locations. The diminishing night time plateau in the downstream direction represents decreased influence of the night time input signal to the diel pattern at a spatial location. Figure 4: Time series of in-stream and hyporheic 17α-TBOH and hydroxy-17α-TBOH concentration at selected spatial locations. Time series of stream and hyporheic concentrations for 17α-TBOH without (left column) and with (right-column) product-to-parent reversion at selected locations. Two typical 24 h cycles are presented for each spatial location. Grey and white shaded regions indicate periods of darkness (reversion dominance in the stream) and daylight (photolysis dominance in the stream), respectively. For cases without-reversion, hyporheic zones alternate between net sources of 17α-TBOH to the stream. The hyporheic zone is a net source of 17α-TBOH when stream concentration is less than hyporheic concentration (that is, during daylight periods when photolysis dominates in the stream). Hyporheic zones are a net sink for in-stream 17α-TBOH when the stream concentration is greater than the hyporheic concentration (typically during periods of darkness). Cases with and without-reversion have similar source-sink behaviour for the first 38 km of transport, but hyporheic zones become persistent sources of 17α-TBOH to the stream beyond this location. In these downstream locations, hyporheic reversion is able to increase in-stream concentrations to nearly 40% of their input concentration in some locations. The diminishing night time plateau in the downstream direction represents decreased influence of the night time input signal to the diel pattern at a spatial location. Full size image Hyporheic zones exhibit time-variable source-sink behaviour Transport and transformation in the stream interact with storage and reversion in the hyporheic zone along the stream, leading to extended resupply of 17α-TBOH to the stream and elevated in-stream concentrations ( Figs 2 and 3 ; Supplementary Movie 1 ). The hyporheic zone acts as a net source of 17α-TBOH to the stream when hyporheic concentrations exceed those in-stream (that is, stream time series above hyporheic time series), and a net sink at times when 17α-TBOH concentrations are lower in the hyporheic zone than in the stream (that is, stream time series below hyporheic time series; Fig. 4 and Supplementary Fig. 2 ). Net source or sink behaviour is defined by the dynamic development of concentration gradients between the stream and hyporheic zone, and the magnitude defined by the exchange rate ( α ) and relative sizes of the stream and hyporheic zone (commonly A s / A ). This dynamic source-sink characteristic is in contrast to definitions of source and sink used for chemical systems without considering product-to-parent reversion, where sinks often indicate irreversible loss, and sources indicate new mass (as opposed to reverted mass) entering the system. The input 17α-TBOH is primarily advected downstream of the input plateau concentration during periods of darkness ( Fig. 4 ). The exchange of water between the stream and hyporheic zones results in a hyporheic concentration always trending towards the in-stream concentrations, but never reaching equilibrium ( Fig. 4 ). The characteristic timescale of exchange is longer than the timescale driving in-channel dynamics (that is, the photoperiod). Exchange of water between the stream and hyporheic zone reduces the amplitude of the diel in-stream concentration time series. Similar hyporheic buffering for stream temperatures varying on a diel basis has been broadly reported. Temporary storage of 17α-TBOH advected downstream during periods of darkness, exchanged into the hyporheic zone, stored temporarily in this domain with no photolysis, and then slowly released back to the stream increases in-stream minimum concentrations of 17α-TBOH. Similarly, the inverse processes occur in daylight and decrease in-stream maximum concentrations. Hyporheic buffering of in-stream concentrations occurs throughout the model domain for both the with- and without-reversion cases. For the case without-reversion, the timing and magnitude of the net source and sink behaviour are solely a reflection of the characteristic timescale of hyporheic exchange relative to the timescale of diel in-stream fluctuations. Large exchange rates and small hyporheic zones cause hyporheic 17α-TBOH concentrations to converge on dynamics identical to those in the stream alone, reducing the buffering effect, while the opposite occurs for the inverse case. For a smaller hyporheic zone and/or faster exchange rate, the stream and hyporheic zone would more closely track in their timeseries. At one extreme, the hyporehic zone would be instantaneously well-mixed with the stream and have minimal impact on the 17α-TBOH timeseries at a location, due to either a small hyporheic zone or extremely rapid exchanges with the stream. Conversely, a low exchange rate would functionally decouple the stream and hyporheic zone. For the case with reversion, the exchange processes described above interact with slowly increasing hyporheic 17α-TBOH concentrations as product-to-parent reversion occurs. After 24 h of transport, daily average in-stream 17α-TBOH concentrations are 12.8 and 0.4% of the input concentrations for the with- and without-reversion cases. Throughout the model domain, particularly the reversion-dominated reach, reversion maintains higher 17α-TBOH concentrations in the stream and hyporheic zone. Increased hyporheic concentrations reduce the net sink function of the hyporheic zone, proportionally increasing its source function ( Fig. 3 ). The magnitude of the net source function is controlled by the rate of 17α-TBOH regeneration relative to the stream-hyporheic zone exchange rate. The source function is minimized wherever the exchange rate removes 17α-TBOH faster than it can be regenerated. In contrast, the without-reversion case loses 10% of the total simulated mass (during the forward photolysis reaction) and then conservatively transports the remaining 90% as hydroxy-17α-TBOH. Although we expect that other attenuation processes affect transport and fate of 17α-TBOH and hydroxy-17α-TBOH, sufficient data characterizing such processes are not available for both species and thus we omitted them from our simulations. Nevertheless, expected behaviour can be described. Reversible sorption-desorption processes would create additional time lags in the temporary storage of 17α-TBOH, increasing buffering of in-stream concentrations (assuming minimal photolysis in the sorbed phase, primarily within the hyporheic zone). Sorption would also represent an irreversible removal of dissolved mass for a permanently bound fraction of the sorbed species. Biotransformation of 17α-TBOH is expected to compete with reversion and reduce concentrations in the stream and/or hyporheic zone. We note, however, that such competing reactions are already integrated into our simulation, with a constant reversion rate and time-variable photolysis rate interacting dynamically though time. On the basis of experimental yields of photoproducts reported by Qu et al . [1] , our model partitions 10% of the photoproducts to non-bioactive species incapable of reversion (for example, species with a substantially modified structure [15] ). This represents a continuous loss of mass over time as product and parent continue to cycle. Additional competing reactions would be expected to simply increase the magnitude of this loss term. If all loss processes are considered first order, the net sum of their reaction rate coefficients would dictate the behaviour of the system. For example, a hyporheic zone with a biotransformation rate for 17α-TBOH larger than its reversion rate would exhibit increased sink behaviour. Periods of net source behaviour are expected to persist even in this case. Finally, characterization of non-linear interactions (for example, those associated with differing behaviour of sorbed and dissolved compounds in the hyporheic zone) is generally lacking and would require increased model complexity. Yield and bioactivity partitioning control ecological risk One benefit of our modelling approach is that we can explore fate and risk scenarios that might otherwise be too difficult to assess via traditional approaches wholly reliant on demanding and expensive analytical measurements. For example, a scenario that complicates risk management for TBA metabolites is that their photoproducts seem to retain some aspects of bioactivity distinct from their parent metabolites [15] . Thus, confining ecological risk considerations only to the known bioactivity of 17α-TBOH would underestimate the ecological hazard posed by the mixture of parent and product bioactivity. This case is not just limited to TBA metabolites, as a growing number of studies demonstrate increased JBA, or total combined bioactivity, attributed to mixtures of parent compounds, metabolites and transformation products. In fact, summed mixture persistence in a network has been termed ‘joint persistence’ where several reactions occur in series to account for the summed persistence of all related compounds [16] , [17] , [18] . Inclusion of bioactivity metrics in a similar framework is a logical extension of this concept. We note that the concept of JBA is beginning to be addressed using regulatory concepts such as ‘predicted no-effect concentrations (PNECs)’ for which mixture bioactivity is the key metric of interest rather than any single concentration of individual constituents [19] , [20] . Indeed, it is probably most logical to move away from regulatory approaches structured around individual constituents in general, and towards biologically driven end points such as those structured within adverse outcome pathways [21] . In some cases, accounting for JBA causes mixtures to exceed PNECs that would not otherwise be met if only the parent compound were considered [22] . Trenbolone metabolites are ideal examples to illustrate mixture bioactivity effects because their product-to-parent reversion dynamics will be key contributors to JBA in affected watersheds. Further, our modelling approach enables us to quantify JBA for 17α-TBOH and its primary photoproduct, hydroxy-17α-TBOH in a stream-hyporheic system at a resolution that is not possible from laboratory experiments or field data alone. We used our model to consider five representative scenarios where bioactivity was apportioned to 17α-TBOH and hydroxy-17α-TBOH through a range of relative potencies (see Methods section). Bioactivity coefficients include subscript ‘17α’ for 17α-TBOH and ‘OH’ for hydroxy-17α-TBOH. The subscripts ‘w’ and ‘w/o’ denote cases with or without product-to-parent reversion, respectively. As a baseline for comparison (Case 1 w/o ), we set a JBA value of 1.0 to represent the bioactivity expected solely by input of 17α-TBOH at the upstream end of the model domain, without considering reversion. This case is considered the baseline for risk assessment because it represents the current regulatory approach to 17α-TBOH fate in the United States (that is, no reversion, no bioactivity attributed to transformation products). For all subsequent cases, we present both absolute JBA and the change in JBA relative to the baseline case ( Fig. 5 ). 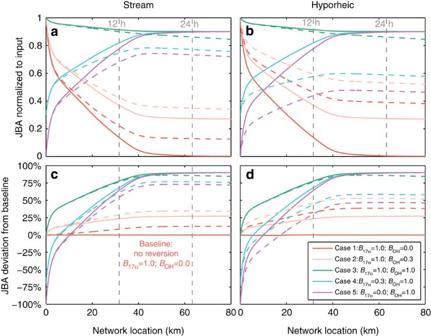Figure 5: Joint bioactivity in the stream and hyporehic zone. In-stream joint bioactivity from simulations of 17α-TBOH and hydroxy-17α-TBOH, calculated by scaling in-stream concentrations by bioactivity coefficients and summing values for both species (top row). Representative cases were calculated with and without-reversion for a range of relative bioactivities, including: Case 1: parent only, Case 2: parent more bioactive than product, Case 3: equal bioactivity, Case 4: product more bioactive than parent and Case 5: product only. Joint bioactivity (JBA) is calculated by scaling concentrations by bioactivity coefficients, and presented as JBA in the stream (left column) and hyporheic zone (right column). In addition, we present the deviation from the baseline conditions where only 17α-TBOH is bioactive and no reversion occurs, the de facto regulatory assumption (bottom row). To demonstrate how the inclusion of increased complexity in chemical processes and bioactive metabolites changes JBA relative to currently regulatory assumptions (only 17α-TBOH is bioactive, no reversion; Case 1 solid lines). In simulations with reversion, the linear decay of bioactivity in the systems with reversion is due to the continued partitioning of 10% of the forward reaction to non-revertible, non-bioactive products. Vertical dashed lines indicate distances for 12 and 24 h of downstream advection in the stream channel. Figure 5: Joint bioactivity in the stream and hyporehic zone. In-stream joint bioactivity from simulations of 17α-TBOH and hydroxy-17α-TBOH, calculated by scaling in-stream concentrations by bioactivity coefficients and summing values for both species (top row). Representative cases were calculated with and without-reversion for a range of relative bioactivities, including: Case 1: parent only, Case 2: parent more bioactive than product, Case 3: equal bioactivity, Case 4: product more bioactive than parent and Case 5: product only. Joint bioactivity (JBA) is calculated by scaling concentrations by bioactivity coefficients, and presented as JBA in the stream (left column) and hyporheic zone (right column). In addition, we present the deviation from the baseline conditions where only 17α-TBOH is bioactive and no reversion occurs, the de facto regulatory assumption (bottom row). To demonstrate how the inclusion of increased complexity in chemical processes and bioactive metabolites changes JBA relative to currently regulatory assumptions (only 17α-TBOH is bioactive, no reversion; Case 1 solid lines). In simulations with reversion, the linear decay of bioactivity in the systems with reversion is due to the continued partitioning of 10% of the forward reaction to non-revertible, non-bioactive products. Vertical dashed lines indicate distances for 12 and 24 h of downstream advection in the stream channel. Full size image For the baseline scenario (Case 1 w/o ; B 17α =1; B OH =0), bioactivity is equal to the concentration of 17α-TBOH, rapidly decreasing in the stream and hyporheic zone upon 17α-TBOH transformation. Daily average JBA in both the stream and hyporheic zone is reduced by 99% at a distance of about 53 km in the network. We take this network location as a key point for comparison between scenarios relative to the baseline. Without-reversion cases approach a plateau beyond this distance, where only dilution by inflows reduces in-stream JBA. For Case 1 w , we found increases in in-stream and hyporheic JBA by 12 and 39% above the baseline at 53 km, respectively. Beyond this network location, all cases with reversion exhibited a persistent JBA fraction in the network, only decreasing by about 1.3% of input JBA per 100 km due to the 10% partitioning to irrevertible, non-bioactive products during each photolysis-reversion cycle. This rate applies to the all source-dominated cases that include reversion. For Case 2 w/o ( B 17α =1; B OH =0.3), where the primary transformation product hydroxy-17α-TBOH retains partial bioactivity, JBA in the stream and hyporheic zone are increased over the baseline scenario by 27% at 53 km. For Case 2 w , increases in JBA are 34 and 53% for the stream and hyporheic zone, respectively. For any cases where B 17α >B OH , concave-up patterns of JBA will be produced in the network, indicating decreasing exposure in the downstream direction and equilibrium favours the less-active form, hydroxy-17α-TBOH. For Case 3 w/o ( B 17α =1; B OH =1), in-stream and hyporheic JBA are about 89% larger than the baseline value at 53 km because the product is substantially more potent than in Case 2. Despite the fact that parent and product are equipotent, input JBA is not perfectly conserved because the stream and hyporheic zone must come into equilibrium. Declines in JBA along the stream reflect the unequal distribution of steroid mass between the stream and hyporheic zone. Elevated JBA levels persist indefinitely in these simulations and are only reduced by competing physical or chemical attenuation processes (for example, dilution by inflow, sorption, biotransformation) in the network. For Case 3 w/o , the 10% partitioning to non-bioactive products occurs only once (that is, no mass undergoes photolysis more than one time), resulting in a constant exposure of JBA through the network after this stream-hyporheic partitioning (horizontal lines in Fig. 5 ). For Case 3 w/o , in-stream and hyporheic JBA are 86% larger than baseline values at 53 km. The slight reduction in JBA compared with Case 3a reflects reverted 17α-TBOH being photolysed and including 10% conversion to stable products over multiple cycles. Cases 4 and 5 reflect systems where product potencies exceed parent potency ( B 17α <B OH ). In each case the input JBA is less than the baseline in relative terms because of the lower potency parent, but JBA rapidly increases in the network as the forward reaction proceeds, exhibiting a characteristic concave-down profile. For Case 4 w/o ( B 17α =0.3; B OH =1), in-stream JBA at 53 km is increased by 88% compared with baseline conditions in both the stream and hyporheic zone. For Case 4 w , increases in JBA over the baseline case in the stream and hyporheic zone are 77 and 58% at 53 km, respectively. For Case 5 w/o ( B 17α =0; B OH =1), JBA in the stream and hyporheic zone is 88% higher than baseline values at 53.3 km. For Case 5 w , increases over baseline are 73 and 47% at 53 km. For cases with B 17α <B OH , representing formation of relatively more potent products, it is not surprising that environmental risk assessment is especially challenging because the location of maximum JBA exposure is not proximal to the release, which necessitates analysis of hydraulic retention times and reaction times. Thus, for cases where products retain some bioactivity, especially where product bioactivity arises from distinct pathways (for example, interacts with a different receptor, different biochemical pathway), it is reasonable to expect maximum impacts at locations distant from contaminant sources. We found that hyporheic exchange and reversion processes increase downstream JBA by 34% in the stream and 53% in the hyporheic zone (Case 2 w ) compared with those estimated by considering only the irreversible forward reaction (Case 1 w/o ). At the time of publication, reliable field sampling and measurement protocols for TBA metabolites and photoproducts have not been established. Thus, the outcomes detailed here are projected based on state-of-the-science laboratory results and numerical models. Compared with a baseline case in which mass is assumed to be fully removed by photolysis occurring rapidly in the stream, these sustained concentrations pose a significant, additional hazard. At a minimum, we believe these results justify the need for revisiting regulatory strategies and considering the use of mixture based PNECs. For endocrine disrupting compounds in general, where source concentrations have been documented at thousands of ng l −1 and impacts demonstrated for tens of ng l −1 or less, these increased concentrations may be ecologically relevant. This modelling also provides a clear demonstration that simplified fate models, such as half-life, are most applicable only proximal to the source. To estimate downstream concentrations or JBA accurately, a new, more complete paradigm is needed. This approach may need to be compound specific, and it must explicitly consider the dominant interacting physical and chemical processes, including formation of transformation products, that govern transport and fate outcomes to avoid underestimation of environmental risk. This issue would be particularly acute for bioactive species with moderate-to-high persistence or potent species known to yield bioactive products, as these compounds may lack sufficient attenuation mechanisms to reduce JBA and associated risk in environmental systems. For compounds where even trace concentrations are ecologically relevant, current risk assessment paradigms are particularly vulnerable to atypical processes such as the reversible transformation driven by physical and/or biogeochemical heterogeneities. For the TBA metabolite simulations presented here, if a PNEC limit is not achieved within the source-dominated reach where rapid decay of JBA dominates, subsequent transport in the reversion-dominated reach will maintain concentrations above the PNEC threshold and JBA will persist at unsafe levels. In systems characterized by product-to-parent reversion, effective removal in the source-dominated reach is critical if a reaction process, such as rapid photo- or biotransformation, dominates expected reductions in environmental risk. Management targeting the source of TBA metabolites or their removal within the source-dominated reach is therefore important to reduce any impact on fluvial ecosystems, rather than relying on naturally occurring attenuation processes farther downstream in the network. Model simulations demonstrate increased persistence for 17α-TBOH and associated JBA in stream systems, where the hyporheic zone becomes a hot-spot for product-to-parent reversion and unexpectedly acts as an important diffuse source of bioactive parent to surface waters. Although 17α-TBOH dynamics are similar in the source-dominated reach for with- and without-reversion cases, where ∼ 60% of removal occurs, reversion subsequently increases removal timescales by a full order of magnitude in the reversion-dominated reach. Finally, depending on relative parent-product potency, which admittedly remains uncertain for most classes of environmental pollutants, we demonstrate the substantial divergence of bioactivity predictions with- and without-reversion, particularly with respect to defining long-term contaminant persistence in the stream. Current regulatory paradigms that focus on individual species fail to address joint persistence and JBA in the environment. Furthermore, those based on representative timescales of an individual reaction are insufficient to characterize ecosystem exposure for chemical systems characterized by product-to-parent reversion and reaction rates driven by heterogeneity in environmental systems (for example, differential reactivity in perpetually dark hyporheic zones versus dynamic forward reactions in streams). The key issue highlighted by this study is demonstrating the potential implications that an atypical or unexpected contaminant characteristic (for example, arising from either environmental reactivity, fate or bioactivity) has on the accuracy of environmental risk assessment. Our simulations demonstrate that conservation of bioactivity between species, especially in systems where physical and chemical heterogeneity interact to control partitioning of parent and transformation products, can represent a critical yet underappreciated component of JBA and subsequent environmental risk. Relative to parent compounds, bioactivity in transformation products and mixtures remains an emerging area of research and is an integral aspect of any transition to systems analysis driven by biological endpoints. Relative environmental risk is a function of yield, potency and persistence. During assessment, unexpectedly high values for any of these parameters represent opportunities for significant underestimation of environmental risk [23] . Accurate understanding of the relationships between these key controls, particularly those efforts that develop insight into potency across biological endpoints, would build more confidence in the effectiveness of any particular environmental risk assessment. Similarly, we demonstrate that, for instances of atypical reaction characteristics and pathways, computational models can play an important role in directing research effort (for example, planning a field campaign) and improving our characterization of the environmental implications of contaminant discharges at systems scales. Numerical model formulation and simulation To quantify the potential impact of product-to-parent reversion on TBA metabolite persistence, we conducted numerical simulations of 17α-TBOH transport and fate in a stream-hyporheic system and compared cases with and without-reversion. The dominant transport processes simulated are advection, dispersion and transient storage in the hyporheic zone [24] . Key assumptions of this model include a well-mixed stream and hyporheic zone at each spatial step, an exponential residence time distribution in the hyporheic zone, and no down-stream transport in the hyporheic zone. We constructed a modified version of this model to represent two interacting species, similar to recent work for the Resazurin-Resorufin tracer [25] . Our 1-D transient storage model simulates transport and fate of 17α-TBOH and its primary photoproduct, hydroxy-17α-TBOH. A version of the computer code use for simulation may be obtained by contacting the corresponding author. For our simulations, we selected physical parameters to represent Fourmile Creek near Ankeny, Iowa, USA, a USGS Field Laboratory for the study of Contaminants of Emerging Concern [26] . The physical system is representative of a third order stream in the Midwestern United States. We assumed a wide, rectangular, plane-bed stream with constant discharge of 500 l s −1 (average annual average discharge 535 to 4,989 l s −1 for water years 2007–2013 at USGS gauge 05485605) and longitudinal slope of 0.1% (average gradient for the first 3.1 km downstream of the USGS gauge site on Fourmile Creek), Darcy-Weisbach friction factor of 0.05. We assigned longitudinal dispersion at 10 −8 m 2 s −1 . We used a 4-point implicit numerical solution scheme to iterate to a steady-state normal depth and velocity for the network [27] . We specified a hyporheic cross-sectional area of 1 m 2 , compared with a stream cross-sectional area of 0.68 m 2 (2 m width, 0.34 m depth). This ratio of hyporheic to stream area (commonly A s / A ) is 1.5. We applied a hyporheic exchange rate of 0.036 h −1 (10 −5 s −1 ). Both hyporheic area and exchange rate are within typically observed ranges for studies using the transient storage model [28] . We simulated a constant-rate input of 5 ng l −1 17α-TBOH at the upstream end of the model domain into the stream. This loading is representative of a low concentration, sustained input due to, for example, leaching from field-applied manure to an agricultural landscape or a leaky manure storage pond. Forward and reversion rate constants were estimated using photolysis and reversion data presented in Qu et al . [1] The reversion rate from hydroxy-17α-TBOH to 17α-TBOH was assumed constant in both the stream and hyporheic zone with a rate constant of 0.02 h −1 . The peak photodegradation rate constant for 17α-TBOH was simulated as 2 h −1 . No photodegradation was assigned to hydroxy-17α-TBOH. The photodegradation rate was simulated as time-dependent, using a half sine-wave to assign a value during a 12 h photoperiod (06:00 to 18:00) and the rate set to zero outside of the photoperiod [29] . We assumed a constant photodegradation rate through the well-mixed water column, given the shallow stream depths simulated. In other systems light penetration through the water column may be controlled by suspended solids concentrations or changes in solar loading in space (for example, shading) and through time (for example, cloud cover). On the basis of observations in Qu et al . [1] , photolysis of 17α-TBOH was assumed to yield 90% revertible products (that is, hydroxy-17α-TBOH) and 10% other products not subject to reversion and assumed non-bioactive (for example, species with a substantially modified structure, such as the 11,12-dialdehyde product we previously reported [15] ). All other parameters were assumed constant in space and time to isolate the effect of the reversion process on results. The model was run continuously until a 24-hour steady-state oscillation was achieved, determined by a change in 24-h peak values of less than 1% between subsequent 24-h cycles at all spatial locations. This spin-up period was at least 480 h for all simulations. Daily maximum and minimum values were extracted from a 24-hour period at this dynamic steady-state. Daily average values were calculated as the arithmetic average of a 24-hour period at this dynamic steady-state. Model variants were completed with- and without-reversion. The model was solved using a Crank-Nicholson solution scheme with spatial steps of 100 m over a 200 km domain and temporal steps of 60 s, after Runkel [30] . Our model represents an improvement in the representation of physical and chemical processes compared with the de facto baseline model used for regulation of 17α-TBOH (photolysis in the stream water only; no hyporheic exchange; no product-to-parent reversion). The model includes product-to-parent reversion in both the stream and hyporheic zone, and time-variable photolysis in the stream. Other attenuation processes (for example, sorption, biodegradation) were not simulated because sufficient data are not available to characterize these processes for 17α-TBOH and its major photoproduct, hydroxy-17α-TBOH. As such, this model represents a system where these attenuation processes are minimized, a worst-case scenario for risk from TBA metabolites. While this model increases the realism of the suite of interacting processes that control the transport and fate of TBA metabolites in the environment, we acknowledge that the assumptions of spatially homogeneous reaction rates and omission of competing attenuation pathways (for example, sorption-desorption, biodegradation, dilution) are limitations of this framework. At this time, there are no published studies characterizing pathways for hydroxy-17α-TBOH other than photolysis. We included only processes for which rate constants and controls are characterized in the literature for both 17α-TBOH and hydroxy-17α-TBOH. Published partitioning coefficients for 17α-TBOH include linear distribution coefficient ( K d ; 2.2–41.1 l kg −1 ) with positive relationships with organic content, pH, clay fraction and cation exchange capacity of the soil [31] , [32] , [33] . Additional available partitioning coefficients include organic carbon normalized (log K oc ; 2.77±0.12), Octanol-water (log K ow ; 2.72±0.02), Hexane-water (log K hw ; −0.114±0.006), chlorophyll-water (log K chw ; 3.36±0.01), cyclohexane-water (log K cyw ; 0.39±0.07) and toluene-water (log K tw ; 1.987±0.01) partitioning coefficients [31] , [33] . First-order biodegradation rates for 17α-TBOH were recently reported as 0.0034, h −1 for 5 °C and 0.0071 to 0.013 h −1 for 20 °C in aerobic batch microcosms [31] . Using these values, we calculate a θ for the Arrhenius equation ranging from 1.038 to 1.072. For typical stream temperatures of 18 °C, biodegradation rate constants are 0.0066–0.011 h −1 (0.33–0.58% of the peak forward reaction rate; 33–58% of the reversion rate). Assuming hyporheic temperatures of 12 °C, biodegradation rate constants are 0.0053–0.0077, h −1 (0.26–0.38% of the peak forward reaction rate; 26–38% of the reversion rate). These values demonstrate the potential rates of other processes controlling 17α-TBOH transport and fate, but are limited in their applicability to our system. These rates were derived from aerobic mesocosms and we do not expect them to be applicable in the typically anaerobic hyporheic zones. To our knowledge, no further data are available about biotransformation rate dependencies on pH, redox conditions, nor other controls for 17α-TBOH. Our model omits any inflows and outflows of water along the domain. Evapotranspiration from the stream could enrich concentrations, though we expect this to be minimal compared with down-stream flux of water in the stream. Finally, we note that gross losses of water from the system to regional groundwater would not effect in-stream concentrations, but would reduce the mass flux of 17α-TBOH and hydroxy-17α-TBOH through the stream and hyporheic zone. Environmental samples of 17α-TBOH and hydroxy-17α-TBOH for model validation are not currently available. Samples collected before discovery of the product-to-parent reversion pathway are extremely limited in their usefulness because interconversion occurs constantly during sample collection and processing, resulting in limited ability to draw meaningful conclusions about field concentrations of 17α-TBOH and hydroxy-17α-TBOH. Indeed, standardized methods to analyse trace concentrations in complex matrices when looking for hydroxylated products and accounting for or eliminating artifacts from reversion do not currently exist. Furthermore, sampling is complicated by the continuous interaction of multiple species between sample collection and processes; transport and storage in the dark would be subject to reversion, while sample prep in the light (as on a laboratory bench) would be subject to photolysis. Calculation of JBA for representative cases To assess the influence of reversion on total bioactivity in the network, we apply a conceptual framework where JBA equals the sum of relative potency multiplied by parent or product concentrations, calculated as: where B is a bioactivity coefficient describing the relative bioactivity of each compound compared with a baseline, (bioactivity per concentration) assumed here as 17α-TBOH, and C is the simulated 24-h mean concentration of each compound normalized to the input concentration of 17α-TBOH. In this study, we use the subscripts 17α for the parent (17α-TBOH), and OH for the product (hydroxy-17α-TBOH). This framework is similar to that used for oestrogenic compounds, where oestrogenicity is commonly reported as additive 17β-estradiol equivalents [34] . At this time, no standard scale akin to oestrogenicity is yet established for androgens, nor are compound-specific bioactivities widely calculated for such compounds. In our study, we consider the de facto regulatory assumption as a baseline case (Case 1; B 17α =1; B OH =0). As relative bioactivities are yet unquantified for TBA metabolites, and to extend our results to other compounds with reversible transformation, we consider four additional cases: Case 2 parent is more bioactive than product (for example, 17α-TBOH and hydroxy-17α-TBOH; B 17α =1; B OH =0.3); Case 3 equal bioactivity of parent and product ( B 17α =1; B OH =1); Case 4 product is more bioactive than parent (for example, reduction of estrone to 17β-estradiol or deconjugation of glucuronides to free steroids; B 17α =0.3; B OH =1) [35] and Case 5 only the product is bioactive ( B 17α =0; B OH =1). These calculations are designed to explore downstream bioactivity exposure as a function of the relative bioactivity of identifiable compounds, one of the emerging cases that must be considered in risk management for compounds’ bioactive products. How to cite this article: Ward, A.S. et al . Coupled reversion and stream-hyporheic exchange processes increase environmental persistence of trenbolone metabolites. Nat. Commun. 6:7067 doi: 10.1038/ncomms8067 (2015).